Efficacy of the β2-adrenergic receptor is determined by conformational equilibrium in the transmembrane region Many drugs that target G-protein-coupled receptors (GPCRs) induce or inhibit their signal transduction with different strengths, which affect their therapeutic properties. However, the mechanism underlying the differences in the signalling levels is still not clear, although several structures of GPCRs complexed with ligands determined by X-ray crystallography are available. Here we utilized NMR to monitor the signals from the methionine residue at position 82 in neutral antagonist- and partial agonist-bound states of β 2 -adrenergic receptor (β 2 AR), which are correlated with the conformational changes of the transmembrane regions upon activation. We show that this residue exists in a conformational equilibrium between the inverse agonist-bound states and the full agonist-bound state, and the population of the latter reflects the signal transduction level in each ligand-bound state. These findings provide insights into the multi-level signalling of β 2 AR and other GPCRs, including the basal activity, and the mechanism of signal transduction mediated by GPCRs. G-protein-coupled receptors (GPCRs) are one of the largest membrane protein families in eukaryotes [1] , and more than 25% of modern drugs target GPCRs [2] . These drugs bind to GPCRs, leading to the induction or inhibition of signal transduction mediated by G-proteins, β-arrestins and various other effectors via GPCRs. Each chemical ligand for a GPCR has a different level of ability to activate or inhibit its target, which is commonly referred to as efficacy, and the ligands are classified according to their efficacies, such as full agonists, partial agonists, neutral antagonists and inverse agonists [3] , [4] . These differences in the efficacies significantly affect the therapeutic properties of the GPCR ligands. In the case of drugs that target β 2 -adrenergic receptor (β 2 AR), a full agonist offers a clinical advantage over a partial agonist in acute severe asthma, although full agonists are capable of causing more adverse effects [5] . Structural analyses of β 2 AR complexed with various ligands are required to clarify the mechanism that determines the ligand efficacies. The crystal structures of β 2 AR have been solved in the forms bound to inverse agonists [6] , [7] , [8] , [9] , [10] , a neutral antagonist [10] , a full agonist [11] and a full agonist with a G-protein [12] or a G-protein-mimicking nanobody [13] (PDB accession codes: 3D4S , 2RH1 , 3PDS , 3SN6 , and 3P0G ). In the structure of the form bound to both a full agonist and a G-protein, the cytoplasmic half of transmembrane 6 (TM6) shifted outward, in comparison with that in the inverse agonist-bound form, and the C-terminal helix of the G-protein was inserted into a cytoplasmic cavity. In addition, the ligand-dependent conformational changes of the solvent-exposed extracellular and intracellular regions were observed in biochemical studies with fluorescent labeling [14] , [15] , [16] , chemical labeling [17] and hydrogen–deuterium exchange techniques [18] , as well as solution NMR analyses using chemical modifications with 13 CH 3 probes [19] . However, the structure of the β 2 AR TM region, which is directly involved in the conformational changes upon ligand binding, has not been examined in the neutral antagonist-bound and partial agonist-bound states. In addition, the crystal structures cannot fully explain the mechanism of the efficacies, including the basal activity [10] . Liu et al . [20] recently incorporated CF 3 probes, which can be observed with high sensitivity and selectivity, into β 2 AR and demonstrated that the 19 F-NMR signals from the CF 3 probe at C265 6.27 (superscripts indicate Ballesteros–Weinstein numbering [21] ) exhibited two components, which are referred to as I and A, and the population of A correlates with the efficacy of each ligand. I and A were structurally characterized by the PRE experiments, which suggested that C327 7.54 is more exposed to solvent in I than in A, in an agonist-bound state [20] . Here we utilized NMR to clarify the conformational diversity of the TM region of β 2 AR in the inverse agonist-bound state, neutral antagonist-bound state, partial agonist-bound states and full agonist-bound state. Our NMR analyses revealed that the methionine residue at position 82 is in a conformational equilibrium between the inverse agonist-bound states and the full agonist-bound state, and the population of the latter reflects the signal transduction level in each ligand-bound state. Preparation and characterization of β 2 AR The E122W/N187E/C265A mutant of β 2 AR (Gly2-Gly365) with an N-terminal FLAG-tag and a C-terminal decahistidine-tag, which exhibited agonist-dependent signalling activities almost identical to the wild type in previous studies [14] , [22] , was expressed in a baculovirus–insect cell expression system. β 2 AR was solubilized by n -dodecyl-β- D -maltopyranoside (DDM), and purified by three chromatography steps, including ligand-affinity chromatography, to more than 95% purity, as judged from SDS–polyacrylamide gel electrophoresis (SDS–PAGE) analyses. The purified β 2 AR is in the formoterol-bound state, because formoterol was added during the elution from the ligand-affinity chromatography. Radioligand-binding assays with an excess amount of [ 3 H]-dihydroalprenolol (DHA), which has a higher affinity for β 2 AR than formoterol [23] , [24] , revealed that more than 80% of the purified β 2 AR retained the DHA-binding activity. We also confirmed that the purified β 2 AR exhibited ligand-dependent conformational changes, by experiments using a fluorescent probe introduced at C265 6.27 (ref. 8 ) ( Fig. 1a,b ). 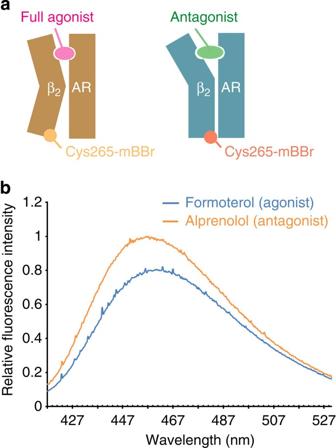Figure 1: Analyses of ligand-dependent conformational changes in β2AR with fluorescent probes. (a) Schematic representation of the fluorescent assay8. A monobromobimane (mBBr) probe is introduced at C2656.27of the β2AR without the C265A mutation (orange). After purification, β2AR is in the formoterol-bound state (brown). By the addition of an excess amount of alprenolol (green), formoterol (magenta) is replaced with alprenolol, resulting in β2AR in the alprenolol-bound state (blue). The receptor conformation shift from an active conformation to an inactive conformation was observed as the increase in the fluorescence intensity of mBBr, due to the change in the local environment. (b) Fluorescence spectra of mBBr-labeled β2AR, in the presence of formoterol (cyan), and after the addition of an excess amount of alprenolol (orange). The fluorescence intensities are normalized to the maximal fluorescence intensity in the alprenolol-bound state. Figure 1: Analyses of ligand-dependent conformational changes in β 2 AR with fluorescent probes. ( a ) Schematic representation of the fluorescent assay [8] . A monobromobimane (mBBr) probe is introduced at C265 6.27 of the β 2 AR without the C265A mutation (orange). After purification, β 2 AR is in the formoterol-bound state (brown). By the addition of an excess amount of alprenolol (green), formoterol (magenta) is replaced with alprenolol, resulting in β 2 AR in the alprenolol-bound state (blue). The receptor conformation shift from an active conformation to an inactive conformation was observed as the increase in the fluorescence intensity of mBBr, due to the change in the local environment. ( b ) Fluorescence spectra of mBBr-labeled β 2 AR, in the presence of formoterol (cyan), and after the addition of an excess amount of alprenolol (orange). The fluorescence intensities are normalized to the maximal fluorescence intensity in the alprenolol-bound state. Full size image Methionine residues are frequently observed in TM3, TM5, and TM6 of GPCR, and these regions exhibit large conformational changes upon activation ( Supplementary Fig. S1 ). β 2 AR possesses nine methionine residues in extracellular loop 1 (ECL1), TM1, TM2, TM4, TM5 and TM6 ( Fig. 2 and Table 1 ), and M82 2.53 ( Supplementary Figs S2 and S3 ), M215 5.54 and M279 6.41 assume distinctly different conformations between the inverse agonist-bound and the full agonist/G-protein-bound crystal structures. Therefore, we utilized the methionine methyl groups to investigate the conformation of the TM region of β 2 AR in various ligand-bound states. Methionine methyl-selective 13 C labeling in the baculovirus–insect cell expression system was accomplished by adding [methyl- 13 C] methionine to methionine-deficient medium. We confirmed that about 90% of the methionine methyl groups in thioredoxin, prepared by the same procedure for β 2 AR, were labeled with 13 C and that the other types of amino-acid residues were not significantly labeled. 1 H- 13 C heteronuclear multiple quantum coherence (HMQC) spectra of the [methyl- 13 C-Met] β 2 AR in the formoterol-bound state were recorded, and those in the carazolol-bound state were recorded by adding an excess amount of carazolol. Degradation of β 2 AR did not occur during the NMR measurements, and the ligand-binding activity remaining after the NMR measurements was about 90% of that of freshly prepared β 2 AR ( Supplementary Fig. S4a and b ). 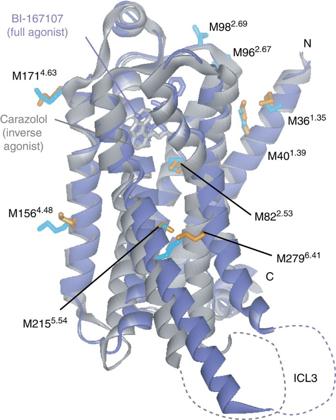Figure 2: Distribution of the methionine residues in the overlaid crystal structures of β2AR. The crystal structure of β2AR with an inverse agonist, carazolol (PDB accession code:2RH1)7, is shown in grey ribbons. Methionine side chains and carazolol are depicted by cyan and grey sticks, respectively. The crystal structure of β2AR with a full agonist, BI-167107, and a G-protein (PDB accession code:3SN6)12is shown in violet ribbons. Methionine sidechains and BI-167107 are depicted by orange and violet sticks, respectively. These structures are overlaid at TM2, and are shown in a side view with the extracellular sides on the upper sides. ICL3 s, which are either substituted with T4 lysozyme or not observed, are shown with dotted lines. Figure 2: Distribution of the methionine residues in the overlaid crystal structures of β 2 AR. The crystal structure of β 2 AR with an inverse agonist, carazolol (PDB accession code: 2RH1 ) [7] , is shown in grey ribbons. Methionine side chains and carazolol are depicted by cyan and grey sticks, respectively. The crystal structure of β 2 AR with a full agonist, BI-167107, and a G-protein (PDB accession code: 3SN6 ) [12] is shown in violet ribbons. Methionine sidechains and BI-167107 are depicted by orange and violet sticks, respectively. These structures are overlaid at TM2, and are shown in a side view with the extracellular sides on the upper sides. ICL3 s, which are either substituted with T4 lysozyme or not observed, are shown with dotted lines. Full size image Table 1 Summary of the differences in β 2 AR methionine resonances in the states with various efficacies. Full size table Spectra of the inverse agonist- and full agonist-bound forms Signals that apparently correspond to the nine methionine residues were observed in the carazolol-bound state ( Fig. 3a ), suggesting that most of the methionine residues were observed, including those in the TM region. Several signals disappeared in the spectrum of the formoterol-bound state ( Fig. 3b ) compared with that in the carazolol-bound state ( Fig. 3a ). 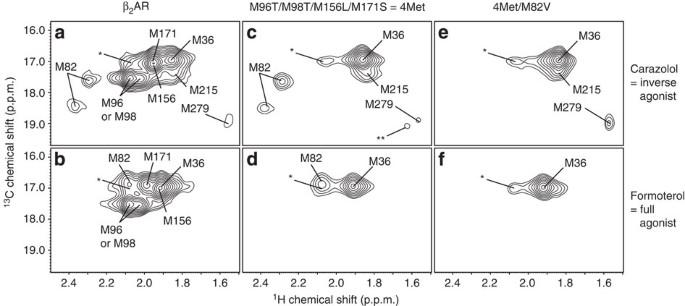Figure 3:1H-13C SOFAST-HMQC spectra of [methyl-13C-Met] β2AR and their assignments. (a,b)1H-13C SOFAST-HMQC spectra of [methyl-13C-Met] β2AR in the carazolol-bound state (a) and in the formoterol-bound state (b). (c,d)1H-13C SOFAST-HMQC spectra of the [methyl-13C-Met] β2AR 4Met mutant in the carazolol-bound state (c) and in the formoterol-bound state (d). (e,f)1H-13C SOFAST-HMQC spectra of the [methyl-13C-Met] β2AR 4Met/M82V mutant in the carazolol-bound state (e) and in the formoterol-bound state (f). The regions with methionine chemical shifts are shown, and the assigned resonances are indicated. The resonances from M40 in the carazolol-bound state, and M40, M215 and M279 in the formoterol-bound state were not observed. Resonances indicated with single asterisk are derived from minor impurity proteins from insect cell membranes, but not from β2AR. Double asterisks are t1noises derived from the intense DDM signal with an1H chemical shift of 1.6–1.7 p.p.m. Figure 3: 1 H- 13 C SOFAST-HMQC spectra of [methyl- 13 C-Met] β 2 AR and their assignments. ( a , b ) 1 H- 13 C SOFAST-HMQC spectra of [methyl- 13 C-Met] β 2 AR in the carazolol-bound state ( a ) and in the formoterol-bound state ( b ). ( c , d ) 1 H- 13 C SOFAST-HMQC spectra of the [methyl- 13 C-Met] β 2 AR 4Met mutant in the carazolol-bound state ( c ) and in the formoterol-bound state ( d ). ( e , f ) 1 H- 13 C SOFAST-HMQC spectra of the [methyl- 13 C-Met] β 2 AR 4Met/M82V mutant in the carazolol-bound state ( e ) and in the formoterol-bound state ( f ). The regions with methionine chemical shifts are shown, and the assigned resonances are indicated. The resonances from M40 in the carazolol-bound state, and M40, M215 and M279 in the formoterol-bound state were not observed. Resonances indicated with single asterisk are derived from minor impurity proteins from insect cell membranes, but not from β 2 AR. Double asterisks are t 1 noises derived from the intense DDM signal with an 1 H chemical shift of 1.6–1.7 p.p.m. Full size image To overcome the severe signal overlaps, we introduced mutations into the solvent- or lipid-exposed methionine residues of β 2 AR (M96 2.67 , M98 2.69 , M156 4.48 and M171 4.63 ), assuming that these mutations would not affect the native folding of β 2 AR. Hereafter, we refer to these residues as 4Met. The HMQC spectra were significantly simplified by introducing the 4Met mutation, because four intense signals disappeared in both the carazolol- and formoterol-bound states ( Fig. 3c,d ). The chemical shifts and signal intensities of the remaining signals did not exhibit significant changes upon introducing the 4Met mutation in both the carazolol- and formoterol-bound states ( Fig. 3a–d ), suggesting that the folding of the 4Met mutant is similar to that of the wild type. For the assignments of the resonances from the methionine in the TM region, we introduced a further mutation into the methionine residue of interest ( Supplementary Fig. S5 ). For example, M82 2.53 was assigned by introducing the M82V mutation into the 4Met mutant ( Supplementary Fig. S5d ). We confirmed that M82V retains the native folding in both the carazolol- and formoterol-bound states, by experiments using a fluorescent probe introduced at C265 6.27 ( Fig. 1b and Supplementary Fig. S6 ). In addition, the M82V mutation does not affect the affinity of the antagonist [ 3 H] DHA to β 2 AR ( Supplementary Fig. S7 ). In the carazolol-bound state, two signals were absent in the spectrum of the M82V mutant, revealing that both of these resonances are from M82 2.53 ( Fig. 3c,e ). Hereafter, we refer to the downfield and upfield resonances from M82 2.53 as M82 D and M82 U , respectively. In the formoterol-bound state, one signal was absent in the spectrum of the M82V mutant, revealing that this resonance is from M82 2.53 ( Fig. 3d,f ). The chemical shifts of the resonance from M82 2.53 in the formoterol-bound state were different from M82 D and M82 U in the carazolol-bound state ( Fig. 4a ). Hereafter, this resonance from M82 2.53 in the full agonist formoterol-bound state is referred to as M82 A . 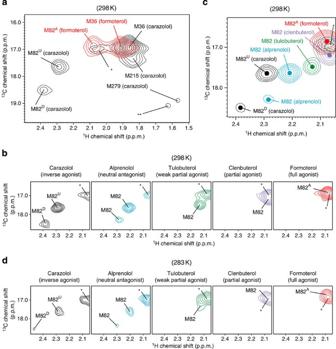Figure 4: The difference in β2AR M822.53resonances in the states with various efficacies. (a) Overlay of the1H-13C SOFAST-HMQC spectra of [methyl-13C-Met] β2AR/4Met at 298 K in the carazolol-bound state (black) and the formoterol-bound state (red). (b)1H-13C SOFAST-HMQC spectra of [α,β,β-2H3-, methyl-13C-Met] β2AR/4Met at 298 K in the carazolol-bound (black), alprenolol-bound (cyan), tulobuterol-bound (green), clenbuterol-bound (violet) and formoterol-bound (red) states. Only the regions with M82 resonances are shown. (c) Overlay of the spectra shown in panelb, with the same colors. The centers of the resonances from M82 are indicated with dots. (d)1H-13C SOFAST-HMQC spectra of [α,β,β-2H3-, methyl-13C-Met] β2AR/4Met at 283 K, with the same colors as in panelb. In panelsa–d, the assigned resonances are indicated with the names of the bound ligands in parentheses (a,c). M82 resonances are indicated with the superscripts used in the main text. Resonances indicated with single asterisk are derived from impurities. Double asterisks are t1noises derived from the intense DDM signal with an1H chemical shift of 1.6-1.7 p.p.m. Figure 4: The difference in β 2 AR M82 2.53 resonances in the states with various efficacies. ( a ) Overlay of the 1 H- 13 C SOFAST-HMQC spectra of [methyl- 13 C-Met] β 2 AR/4Met at 298 K in the carazolol-bound state (black) and the formoterol-bound state (red). ( b ) 1 H- 13 C SOFAST-HMQC spectra of [α,β,β- 2 H 3 -, methyl- 13 C-Met] β 2 AR/4Met at 298 K in the carazolol-bound (black), alprenolol-bound (cyan), tulobuterol-bound (green), clenbuterol-bound (violet) and formoterol-bound (red) states. Only the regions with M82 resonances are shown. ( c ) Overlay of the spectra shown in panel b , with the same colors. The centers of the resonances from M82 are indicated with dots. ( d ) 1 H- 13 C SOFAST-HMQC spectra of [α,β,β- 2 H 3 -, methyl- 13 C-Met] β 2 AR/4Met at 283 K, with the same colors as in panel b . In panels a–d , the assigned resonances are indicated with the names of the bound ligands in parentheses ( a , c ). M82 resonances are indicated with the superscripts used in the main text. Resonances indicated with single asterisk are derived from impurities. Double asterisks are t 1 noises derived from the intense DDM signal with an 1 H chemical shift of 1.6-1.7 p.p.m. Full size image The resonances from M215 5.54 and M279 6.41 in the carazolol-bound state were also assigned using the 4Met-based mutants ( Supplementary Fig. S5e,f ). The spectra of the mutants for M215 5.54 and M279 6.41 in the formoterol-bound state were not significantly different from those without these mutations, suggesting that the resonances from M215 5.54 and M279 6.41 were not observed in the formoterol-bound state ( Fig. 4a ). M82 in the states bound with antagonist and partial agonists To investigate the structures of the TM region in the neutral antagonist-bound and partial agonist-bound states, the HMQC spectra of the 4Met mutant labeled with methyl- 13 C-Met were recorded in the state bound with the neutral antagonist, alprenolol, and in those bound with the partial agonists, tulobuterol and clenbuterol ( Fig. 4b,c ). Alprenolol does not alter the basal activity of β 2 AR [16] , [19] . Clenbuterol reportedly has higher efficacy than tulobuterol [24] ( Supplementary Table S1 ). The tulobuterol- and clenbuterol-bound states were achieved by extensive washing with these ligands on cobalt-affinity resin after the ligand-affinity purification steps. The alprenolol-bound state was attained by adding an excess amount of alprenolol over clenbuterol. As a result, in the alprenolol-bound state, a major and a minor resonance that slightly shifted from M82 U and M82 D , respectively, were observed ( Fig. 4b,c ). In both the tulobuterol- and clenbuterol-bound states, a signal was observed at a chemical shift between M82 U and M82 A , and the chemical shifts in the tulobuterol-bound state were closer to those of M82 U ( Fig. 4b,c ). To examine whether the resonances from M82 2.53 in the ligand-bound states undergo conformational exchange, we also recorded the spectra at a lower temperature, 283 K ( Fig. 4d and Supplementary Fig. S8 ). As a result, the resonances from M82 2.53 in the tulobuterol- and clenbuterol-bound states significantly shifted away from M82 U , and the M82 A resonance in the formoterol-bound state slightly shifted away from M82 U at 283 K ( Fig. 4d and Supplementary Fig. S8a–c ), whereas the resonances from the methyl groups of tulobuterol and clenbuterol did not shift ( Supplementary Fig. S8d,e ). In the spectra of β 2 AR with lower concentrations of clenbuterol and tulobuterol, the signals were observed at the same chemical shifts as those at higher ligand concentrations ( Supplementary Fig. S9 ), suggesting that the NMR signals are not significantly affected by the exchange between the free and bound states or non-specific effect of the ligands, because β 2 AR is only in the ligand-bound state under the present solution conditions. This is consistent with the estimation of the bound population of β 2 AR by the ligand concentration of the NMR samples and the reported affinities of the ligands ( Supplementary Table S1 ). Signals from the residues except for M82 The resonances from M215, which is in the intracellular side of TM5, in the states with carazolol, alprenolol, tulobuterol, clenbuterol and formoterol are shown in Fig. 5a,b . M215 exhibited single resonance in the carazolol-, alprenolol-, tulobuterol- and clenbuterol-bound states ( Fig. 5a,b ). The chemical shifts in the alprenolol- and tulobuterol-bound states were between those in the carazolol- and clenbuterol-bound states, and the chemical shifts in the alprenolol-bound state were closer to those in the carazolol-bound state. The intensities were in the following order: carazolol-bound state >alprenolol-bound state >tulobuterol-bound state >clenbuterol-bound state and the resonances from M215 were not observed in the formoterol-bound state ( Table 1 ). As the temperature was lowered from 298 K to 283 K, the M215 resonances in the carazolol- and alprenolol-bound states shifted towards that in the carazolol-bound state ( Supplementary Fig. S10 ). The chemical shifts and intensities of the resonances from M279, which is in the intracellular side of TM6, also exhibited similar bound ligand-dependent changes ( Fig. 5c ). 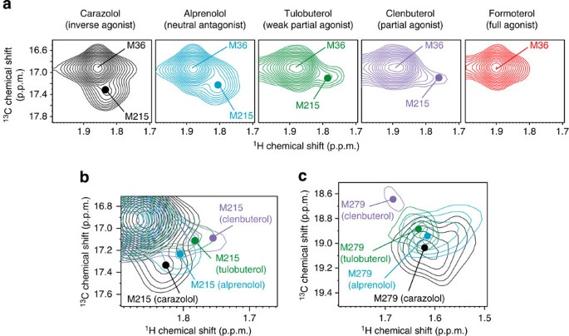Figure 5: The difference in β2AR M2155.54or M2796.41resonances in the states with various efficacies. (a)1H-13C SOFAST-HMQC spectra of [α,β,β-2H3-, methyl-13C-Met] β2AR/4Met at 298 K in the carazolol-bound (black), alprenolol-bound (cyan), tulobuterol-bound (green), clenbuterol-bound (violet) and formoterol-bound (red) states. Only regions with M36 and M215 resonances are shown. (b) Overlay of the spectra shown in panela, except for the formoterol-bound state, with the same colors. In panelb, only the regions with M215 resonances are shown. The centers of the resonances from M215 are indicated with dots. (c) Overlay of the regions with M279 resonances of the1H-13C SOFAST-HMQC spectra of [α,β,β-2H3-, methyl-13C-Met] β2AR/4Met at 298 K in the carazolol-bound (black), alprenolol-bound (cyan), tulobuterol-bound (green) and clenbuterol-bound (violet) states. The centers of the resonances from M279 are indicated with dots. The line shapes of the M279 resonances are distorted due to the overlaps with the t1noises derived from the intense DDM signal with an1H chemical shift of 1.6-1.7 p.p.m. Figure 5: The difference in β 2 AR M215 5.54 or M279 6.41 resonances in the states with various efficacies. ( a ) 1 H- 13 C SOFAST-HMQC spectra of [α,β,β- 2 H 3 -, methyl- 13 C-Met] β 2 AR/4Met at 298 K in the carazolol-bound (black), alprenolol-bound (cyan), tulobuterol-bound (green), clenbuterol-bound (violet) and formoterol-bound (red) states. Only regions with M36 and M215 resonances are shown. ( b ) Overlay of the spectra shown in panel a , except for the formoterol-bound state, with the same colors. In panel b , only the regions with M215 resonances are shown. The centers of the resonances from M215 are indicated with dots. ( c ) Overlay of the regions with M279 resonances of the 1 H- 13 C SOFAST-HMQC spectra of [α,β,β- 2 H 3 -, methyl- 13 C-Met] β 2 AR/4Met at 298 K in the carazolol-bound (black), alprenolol-bound (cyan), tulobuterol-bound (green) and clenbuterol-bound (violet) states. The centers of the resonances from M279 are indicated with dots. The line shapes of the M279 resonances are distorted due to the overlaps with the t 1 noises derived from the intense DDM signal with an 1 H chemical shift of 1.6-1.7 p.p.m. Full size image The HMQC spectra of the β 2 AR without the 4Met mutation were also recorded in the state bound with alprenolol, tulobuterol and clenbuterol, as well as carazolol and formoterol ( Supplementary Fig. S11 ). As a result, the chemical shift changes observed for the β 2 AR without the 4Met mutation were almost identical to those for the 4Met mutant, although the M82 resonances partially overlapped with the resonances from M96 or M98. Therefore, we can rule out the effect of the 4Met mutation on the efficacy in each ligand-bound state. The differences in the other methionine resonances in each ligand-bound state are summarized in Fig. 6 and Table 1 . The resonances from M36, M96/M98, M156 and M171 exhibited only small chemical shift differences in each ligand-bound state ( Fig. 6 and Table 1 ). 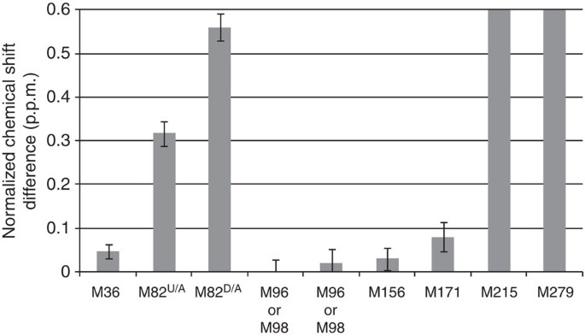Figure 6: Normalized chemical shift differences of the methionine methyl resonances between the carazolol- and formoterol-bound states. Normalized chemical shift differences,Δδ, were calculated by the equationΔδ={(Δδ1H)2+(Δδ13C/3.5)2}0.5. The normalization factor (3.5) is the ratio of the s.d. of the methionine methyl1H and13C chemical shifts, deposited in the Biological Magnetic Resonance Data Bank (http://www.bmrb.wisc.edu/). The error values were calculated by the formula {Δδ1H·R1H+Δδ13C·R13C/(3.5)2}/Δδ, whereR1HandR13Care the digital resolutions in p.p.m. in the1H and13C dimensions, respectively. The number of replicates is greater than two. For M82, both of theΔδs between M82Uand M82A(M82U/A), and M82Dand M82A(M82D/A) were calculated. For M215 and M279, we could not calculate theΔδs between the carazolol- and formoterol-bound states, because these resonances were not observed in the formoterol-bound state, althoughΔδs between the carazolol- and clenbuterol-bound states, which should be smaller than those between the carazolol- and formoterol-bound states, were >0.1 p.p.m. Figure 6: Normalized chemical shift differences of the methionine methyl resonances between the carazolol- and formoterol-bound states. Normalized chemical shift differences, Δδ , were calculated by the equation Δδ ={( Δδ 1H ) 2 +( Δδ 13C /3.5) 2 } 0.5 . The normalization factor (3.5) is the ratio of the s.d. of the methionine methyl 1 H and 13 C chemical shifts, deposited in the Biological Magnetic Resonance Data Bank ( http://www.bmrb.wisc.edu/ ). The error values were calculated by the formula { Δδ 1H · R 1H + Δδ 13C · R 13C /(3.5) 2 }/ Δδ , where R 1H and R 13C are the digital resolutions in p.p.m. in the 1 H and 13 C dimensions, respectively. The number of replicates is greater than two. For M82, both of the Δδ s between M82 U and M82 A (M82 U/A ), and M82 D and M82 A (M82 D/A ) were calculated. For M215 and M279, we could not calculate the Δδ s between the carazolol- and formoterol-bound states, because these resonances were not observed in the formoterol-bound state, although Δδ s between the carazolol- and clenbuterol-bound states, which should be smaller than those between the carazolol- and formoterol-bound states, were >0.1 p.p.m. Full size image Different spectrum patterns from the M82 2.53 methyl group are observed, depending on the efficacy of the bound ligand: the resonances of M82 U and M82 D in the inverse agonist-bound state, two resonances with slightly different chemical shifts from M82 U and M82 D in the neutral antagonist-bound state, one resonance with a chemical shift between M82 U and M82 A in the partial agonist-bound states and the resonance of M82 A in the full agonist-bound state ( Fig. 4b–d ). Based on the comparison between the β 2 AR crystal structures in the forms bound with an inverse agonist and with both a full agonist and a G-protein, the following structural mechanism for GPCR activation was proposed [13] : full agonists induce a conformational change of S207 5.46 and a subsequent rearrangement of the interactions between the TM helices in the middle of the TM region; the inward shifts of TM5 and TM7 at P211 5.50 and N318 7.45 , respectively, and the axial shifts of TM3 and TM6 at I121 3.40 and F282 6.44 , respectively, resulting in a large outward movement of the cytoplasmic half of TM6 ( Supplementary Fig. S2 ). The M82 2.53 side chain also exhibits a dramatic conformational change upon activation, and this conformational change strongly correlates with the rearrangement of the interactions between I121 3.40 and F282 6.44 ( Supplementary Fig. S3 ), via the inward shift of TM7 at Y316 7.43 and S319 7.46 and the axial shift of TM3 at C116 3.35 ( Supplementary Fig. S2 ). Therefore, the side-chain conformation of M82 2.53 would be sensitive to the activation state of β 2 AR. On the other hand, M82 2.53 is 5–8 Å away from the conserved β-OH groups of the β 2 AR ligands, and is not directly involved in the ligand binding. Therefore, the resonances from M82 2.53 would be less affected by the direct interactions with ligands. This is supported by further observation that the affinity of the antagonist [ 3 H] DHA for the 4Met/M82V mutant was almost identical to that for the 4Met mutant ( Supplementary Fig. S7 ). The 13 C and 1 H chemical shifts of the methionine methyl signals are reportedly affected by its side-chain conformation and the local environments, including the ring current effects from the neighbouring aromatic rings, respectively [25] , [26] , [27] . Based upon the crystal structures of β 2 AR, we propose that the M82 U and M82 D signals correspond to the inactive states that cannot directly activate G-proteins, and the M82 A signal corresponds to the active state that can interact with G-proteins ( Supplementary Discussion ). Therefore, the differences between the conformations corresponding to M82 U and M82 D are found in a limited region close to the ligand-binding site. In contrast, the differences between the conformations corresponding to M82 U/D and M82 A are found in the TM region. Hereafter, we refer to these conformations corresponding to M82 U , M82 D and M82 A as the M82 U conformation, the M82 D conformation and the M82 A conformation, respectively. Previous comprehensive analyses of efficacies in various ligands revealed that the efficacies increase in the following order [24] : an inverse agonist, carazolol; a neutral antagonist, oxprenolol, which is an analogue of alprenolol; a weak partial agonist tulobuterol; a partial agonist, clenbuterol; and a full agonist, formoterol ( Supplementary Table S1 ). In the neutral antagonist-bound and partial agonist-bound states, the M82 2.53 resonances exhibited chemical shifts between M82 U and M82 A in an efficacy-dependent manner ( Fig. 4c ). The resonances from M82 2.53 in the partial agonist-bound states shifted towards M82 A as the temperature was lowered from 298 K to 283 K ( Supplementary Fig. S8a,b ). The temperature-dependent shifts, together with the chemical shifts in an efficacy-dependent manner, suggest that β 2 AR exists in equilibrium between the M82 U and M82 A conformations in the partial agonist-bound states, with faster exchange rates than the chemical shift difference. The observation of two resonances from M82 2.53 in the carazolol- and alprenolol-bound states suggests that β 2 AR exists in equilibrium between the M82 D and M82 U conformations in the inverse agonist- and neutral antagonist-bound states, with slower exchange rates than the chemical shift difference. The two resonances from M82 2.53 in the alprenolol-bound state were closer to M82 A than those in the carazolol-bound state, suggesting that the minor population of the M82 A conformation, in equilibrium with the M82 U conformation, would also exist in this state, as supported by the simulation of M82 2.53 resonances ( Supplementary Discussion ). The incomplete linearity of the efficacy-dependent chemical shift change might be derived from another equilibrium within the M82 A conformation. Similar phenomena were also observed for the M215 and M279 resonances. The M215 and M279 resonances exhibited the chemical shifts and intensities in an efficacy-dependent manner ( Fig. 5 and Table 1 ), and these resonances shifted towards those in the carazolol-bound state at lower temperature ( Supplementary Fig. S10a and b ). The simulations of these resonances, with the same parameter as that of the M82 resonances, were in good agreement with the observed spectra ( Supplementary Discussion ). Therefore, the efficacy-dependent conformational equilibrium between the M82 D/U and M82 A conformations observed for M82 2.53 accompanies large conformational changes on TM5 and TM6. Based on the above structural interpretation of the resonances from M82, we propose the following signal regulation mechanism. In the full agonist formoterol-bound state, most of the β 2 AR molecules assume the active conformation ( Fig. 7a ). In the partial agonist tulobuterol- and clenbuterol-bound states, β 2 AR exists in an equilibrium between the inactive and active conformations ( Fig. 7b ), and the populations of the two conformations determine the efficacies. This is in good agreement with the significant, but reduced, efficacy for tulobuterol and clenbuterol [24] . In the neutral antagonist alprenolol-bound state, β 2 AR exists in equilibrium between two major inactive conformations, which are different only in the region close to the ligand-binding site, and one minor active conformation ( Fig. 7c ). The weak basal activity is due to the existence of the minor M82 A conformation. In the inverse agonist-bound state, β 2 AR exists in equilibrium between the two locally different inactive conformations ( Fig. 7d ). Considering that the basal activity partly remained even in the carazolol-bound state [16] , [24] , there may be a minor population of the M82 A conformation in this state, in an equilibrium with one of the inactive conformations. 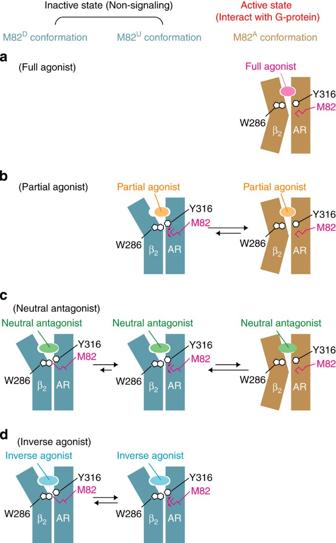Figure 7: A proposed mechanism for the differences in the efficacy of β2AR for different ligands. β2AR adopts three conformations with different M822.53environments; the M82Aconformation induces signalling, whereas the M82Uand M82Dconformations do not. M82Uand M82Aconformations are largely different on TM5 and TM6, whereas the differences between M82Dand M82Uconformations are localized in the region close to the ligand-binding site. (a) In the full agonist formoterol-bound state, β2AR adopts mostly the M82Aconformation, exhibiting almost full efficacy of β2AR. (b) In the partial agonist clenbuterol- and tulobuterol-bound states, β2AR exists in equilibrium between the M82Aand M82Uconformations, exhibiting the significant signaling with reduced efficacies. In the tulobuterol-bound state, where the efficacy is lower than that of the clenbuterol-bound state, the populations of the M82Uconformation are larger. (c) In the neutral antagonist alprenolol-bound state, β2AR adopts mostly the M82Uand M82Dconformations, in equilibrium with a small population with the M82Aconformation. The presence of the small population with the M82Aconformation accounts for the basal activity of β2AR. (d) In the inverse agonist carazolol-bound state, β2AR exists in equilibrium between the M82Uand M82Dconformations, exhibiting the inhibition of basal activities described in panelc. Figure 7: A proposed mechanism for the differences in the efficacy of β 2 AR for different ligands. β 2 AR adopts three conformations with different M82 2.53 environments; the M82 A conformation induces signalling, whereas the M82 U and M82 D conformations do not. M82 U and M82 A conformations are largely different on TM5 and TM6, whereas the differences between M82 D and M82 U conformations are localized in the region close to the ligand-binding site. ( a ) In the full agonist formoterol-bound state, β 2 AR adopts mostly the M82 A conformation, exhibiting almost full efficacy of β 2 AR. ( b ) In the partial agonist clenbuterol- and tulobuterol-bound states, β 2 AR exists in equilibrium between the M82 A and M82 U conformations, exhibiting the significant signaling with reduced efficacies. In the tulobuterol-bound state, where the efficacy is lower than that of the clenbuterol-bound state, the populations of the M82 U conformation are larger. ( c ) In the neutral antagonist alprenolol-bound state, β 2 AR adopts mostly the M82 U and M82 D conformations, in equilibrium with a small population with the M82 A conformation. The presence of the small population with the M82 A conformation accounts for the basal activity of β 2 AR. ( d ) In the inverse agonist carazolol-bound state, β 2 AR exists in equilibrium between the M82 U and M82 D conformations, exhibiting the inhibition of basal activities described in panel c . Full size image Two mechanisms have been proposed for the partial efficacies in the partial agonist-bound states: the equilibrium between the active and inactive states, and the distinct conformation of the partial agonist-bound state from those of both the active and inactive states [3] , although there have been no experimental evidence for them. The chemical shifts of the M82 2.53 resonances in the efficacy-dependent and the temperature-dependent manner in the partial agonist-bound states suggest the equilibrium between the active and inactive states. The M82 D resonance was observed only in the inverse agonist- and neutral antagonist-bound states, and the intensity of the M82 D resonance is higher in the inverse agonist-bound state than in the neutral antagonist state. In addition, the 13 C chemical shifts of M82 U and M82 D suggest that the M82 U conformation flexibly adopts both the trans and gauche conformations, whereas the M82 D conformation mainly adopts the trans conformation ( Supplementary Discussion ); therefore, the M82 D conformation may be more rigid than the M82 U conformation. It is thus tempting to speculate that the M82 D conformation is more refractory to shifting to the activated state than the M82 U conformation, and the higher population of the M82 D conformation in the inverse agonist-bound state causes the inhibition of the basal activity. The resonances from M215 5.54 and M279 6.41 , which are located on the cytoplasmic side of the TM region, were not observed in the formoterol-bound state, suggesting that these signals were broadened due to the conformational exchange between the multiple conformations in the formoterol-bound state. The multiple conformations on the cytoplasmic side of the TM region in the full agonist-bound state may be effective for interacting with various effectors in the conformational selection manners [20] . A number of β 2 AR ligands have been shown to impart differing degrees of signalling in G-protein and arrestin pathways, a phenomenon called 'functional selectivity' or 'biased signalling' [20] , [28] , [29] , [30] , [31] , [32] . The biased signalling is important for both understanding the functions of GPCRs and drug development, and it is quite interesting to investigate the conformations of β 2 AR in the biased ligand-bound states. Although biased signalling was not reported for the ligands chosen in this study [20] , the biased signalling may be due to the diversity of the conformational dynamics in the cytoplasmic side of the TM region in each ligand-bound state. The conformational differences between the crystal structures of β 2 AR were also basically observed in those of adenosine A 2A receptor and rhodopsin [33] , [34] , [35] . In addition, methionine residues are highly abundant in TM3, TM5 and TM6, as described above ( Supplementary Fig. S1 ), and can be observed without any chemical modification. Therefore, the methionine 1 H- 13 C resonances, including Met 2.53 , are broadly applicable for the analyses of the bound ligand efficacy-dependent conformational differences in various GPCRs. Reagents and buffers All reagents were from Nacalai Tesque, unless otherwise noted. The [α,β,β- 2 H 3 , methyl- 13 C] methionine was prepared by the enzymatic deuteration of [methyl- 13 C] methionine (ISOTEC or Cambridge Isotope Laboratories) with Escherichia coli cystathionine-γ-synthase, as previously described [36] . Alprenolol-cysteamine (AlpC) was synthesized as previously described [22] . Affi-gel/AlpC was prepared by coupling 5 mg ml −1 AlpC solution with Affi-gel10 (Bio-Rad) in a dimethyl sulfoxide (DMSO, Dojindo) solution, according to the manufacturer's instructions. Carazolol (Wako Chemicals) and formoterol (Sigma) were solubilized at 100 mM in DMSO-d 6 (ISOTEC), and diluted with buffers. Tulobuterol (Wako Chemicals) was solubilized at 400 mM in methanol-d 4 (ISOTEC), and diluted with buffers. Alprenolol (Sigma) and clenbuterol (Wako Chemicals) were solubilized at 100 mM in D 2 O (Cambridge Isotope Laboratories), and diluted with buffers. Generation of β 2 AR recombinant baculovirus The complementary DNA fragment encoding human β 2 AR (Gly2-Gly365), with an N-terminal FLAG-tag (DYKDDDAA) and a C-terminal decahistidine-tag was amplified by PCR and cloned into the pFastBac1 vector (Invitrogen) via the Bam HI- Xba I sites. The sequence encoding the gp64 signal sequence was amplified from the pBAC-6 vector (Novagen), and placed immediately 5′ to the FLAG-tag. Mutations were introduced by either a QuikChange site-directed mutagenesis kit or a QuikChange multi site-directed mutagenesis kit (Stratagene). E122W, N187E and C265A mutations were introduced in all constructs, unless otherwise stated. Sf9 cells (Invitrogen) were routinely maintained at 27 °C in Grace's supplemented medium (GIBCO) containing 10% fetal bovine serum (Biowest), 0.1% Pluronic F-68 (GIBCO), 50 international units per ml penicillin, 50 μg ml −1 streptomycin and 0.125 μg ml −1 amphotericin B. Recombinant baculoviruses were generated and amplified with the Bac-to-Bac system (Invitrogen), according to the manufacturer's instructions. Expression and purification of β 2 AR The expresSF+ cells (SF+ cells, Protein Sciences) were routinely maintained at 27 °C in 100 ml Sf-900 II serum-free medium (GIBCO), with 50 international units per ml penicillin, 50 μg ml −1 streptomycin and 0.125 μg ml −1 amphotericin B, in a 250 ml Erlenmeyer flask (Corning) on an orbital shaker (130 r.p.m.). For the expression of [methyl- 13 C-Met] β 2 AR, SF+ cells in Sf-900 II medium were centrifuged at 200 g , and resuspended in methionine-depleted ESF921 medium (Expression Systems), at about 2×10 6 cells per ml. For the expression of non-labeled β 2 AR, Sf-900 II medium was utilized instead of the methionine-depleted ESF921 medium. The cells were inoculated with the high-titer virus stock (40 ml per 1 l of cells). After 16 h post infection, 200 mg l −1 [methyl- 13 C] methionine was added. Cells were harvested 48 h post infection by centrifugation at 1,000 g , and the resulting cell pellets were stored at −80 °C. For the expression of [α,β,β- 2 H 3 -, methyl- 13 C-Met] β 2 AR, 200 mg l −1 [α,β,β- 2 H 3 , methyl- 13 C] methionine was added instead of [methyl- 13 C] methionine. All of the following procedures were either performed on ice or in the cold room (4 °C). The cell pellet from 0.8 l of cell culture was re-suspended in 100 ml buffer A (50 mM Tris, pH 8.0, 100 mM NaCl, 1 mM EDTA, 1 mM 4-(2-aminoethyl) benzenesulfonyl fluoride hydrochloride (AEBSF), 10 μM leupeptin hemisulfate (Peptide Institute), 14 μM E-64 (Peptide Institute), 0.3 μM aprotinin (Wako Chemicals)). The cells were disrupted by nitrogen cavitation (Parr Bomb) under 600 p.s.i. for 30 min. The cell lysate was centrifuged at 800 g for 10 min, and the resulting supernatant was centrifuged at 100,000 g for 60 min. The membrane pellet was suspended in buffer B (20 mM HEPES, pH 7.2, 150 mM NaCl, 15% (v/v) glycerol, 100 μM AEBSF, 10 μM leupeptin hemisulfate, 14 μM E-64) and was stored at −80 °C. The membranes obtained from 0.8 l of cell culture were solubilized in 40 ml of buffer B, supplemented with 1% n -dodecyl-β- D -maltopyranoside (DDM, Dojindo) for 4 h, and were then centrifuged at 100,000 g for 30 min. The supernatant was batch incubated overnight with 1 ml of TALON metal affinity resin (Clontech). The resin was washed with 30 ml of buffer B, supplemented with 0.1% DDM and 20 mM imidazole. The protein was eluted with 8 ml of buffer B, supplemented with 0.1% DDM and 200 mM imidazole. For the ligand-affinity chromatography, the eluate from the TALON affinity resin was batch incubated for 4 h with 0.5 ml of Affi-gel/AlpC. The resin was washed with 10 ml of buffer B, and supplemented with 0.1% DDM. The protein was eluted overnight by a batch incubation of the resin with 5 ml of buffer B, supplemented with 0.1% DDM and 1 mM formoterol. For the concentration and the ligand exchange of β 2 AR, a second TALON affinity step was performed after the ligand-affinity chromatography. The eluate from the ligand-affinity chromatography was batch incubated for 1 h with 0.5 ml of TALON resin. The resin was washed with 5 ml of buffer B, supplemented with 0.1% DDM and 100 μM formoterol. The ligand exchange from formoterol to clenbuterol or tulobuterol was accomplished by further washing of the resin for about 3 h, with 50 ml of buffer B, supplemented with 0.1% DDM and 1 mM ligands (clenbuterol or tulobuterol). The protein was eluted with 1 ml of buffer B, supplemented with 0.08% DDM, 200 mM imidazole and the ligands (100 μM formoterol, 1 mM clenbuterol or 1 mM tulobuterol). The eluate from the second TALON affinity step was concentrated using a centrifugal filter device (AmiconUltra-4, 30 kDa molecular weight cutoff, Millipore), while simultaneously exchanging the buffer to buffer C (20 mM sodium phosphate, pH 7.1, H 2 O/D 2 O = 1/99), supplemented with the ligands (100 μM formoterol, 1 mM clenbuterol or 1 mM tulobuterol). In total, 50–400 μg of β 2 AR and its mutants were obtained per 0.8 l of insect cell culture. NMR experiments All of the spectra were recorded with a Bruker Avance 800 spectrometer equipped with a cryogenic probe, and were processed by Topspin 2.1. (Bruker). The assignment of the methionine methyl 1 H- 13 C resonances of β 2 AR was accomplished by the following procedure. 1 H- 13 C SOFAST-HMQC spectra [37] and 1 H- 13 C HMQC spectra with echo/anti-echo gradient coherence selections [38] were recorded for 5–40 μM [methyl- 13 C-Met] β 2 AR and its mutants in buffer C, supplemented with 100 μM formoterol at 298 K. After the NMR experiments, carazolol was added to a final concentration of 500 μM, and 1 H- 13 C SOFAST-HMQC spectra and 1 H- 13 C HMQC spectra with echo/anti-echo gradient coherence selections were recorded at 298 K, for the assignment of the methionine methyl 1 H- 13 C resonances in the carazolol-bound states. 1 H- 13 C HMQC spectra with echo/anti-echo gradient coherence selections were utilized to discriminate the methionine resonances from the t 1 noises derived from the intense DDM signals in the 1 H- 13 C SOFAST-HMQC spectra. The structures of β 2 AR in the various ligand-bound states were investigated by the following procedure. 1 H- 13 C SOFAST-HMQC spectra were recorded for 20 μM [α,β,β- 2 H 3 -, methyl- 13 C-Met] β 2 AR 4Met mutant and 40 μM [methyl- 13 C-Met] β 2 AR in buffer C, supplemented with ligands (100 μM formoterol, 1 mM clenbuterol or 1 mM tulobuterol) at 283 K and 298 K. After the NMR experiments in the formoterol- and clenbuterol-bound states, carazolol and alprenolol were added to final concentrations of 500 μM and 1 mM, respectively, and 1 H- 13 C SOFAST-HMQC spectra were recorded at 283 K and 298 K. 1 H- 13 C SOFAST-HMQC spectra were recorded by excitation with a 4-ms PC9 120 degree pulse [39] and the inversion of a 2-ms Q3 180 degree pulse [40] . For all of the spectra, the spectral widths were set to 12,800 Hz and 4,800 Hz for the 1 H and 13 C dimensions, respectively, and the inter-scan delays were set to 1 s. For the spectra recorded at 298 K in Supplementary Figs S5e-h , 1,024×128 complex points were recorded, and 256 scans/FID gave rise to an acquisition time of 10 h for each spectrum. For the other spectra recorded at 298 K, 1,024×256 complex points were recorded, and 128 scans/FID gave rise to an acquisition time of 10 h for each spectrum. For the spectra recorded at 283 K, 1,024×192 complex points were recorded and 256 scans/FID gave rise to an acquisition time of 15 h for each spectrum. All the spectra were referenced with 3-(trimethylsilyl)-1-propanesulfonic acid sodium salt in both 1 H and 13 C dimensions. How to cite this article: Kofuku Y. et al . Efficacy of the β 2 -adrenergic receptor is determined by conformational equilibrium in the transmembrane region. Nat. Commun. 3:1045 doi: 10.1038/ncomms2046 (2012).